A polyaromatic molecular tube that binds long hydrocarbons with high selectivity Long hydrocarbon chains are essential components of biomolecules used for structure and function in living organisms. The selective recognition and effective binding of hydrocarbons within synthetic host compounds are problematic owing to their conformational flexibility and the lack of specific binding sites. Here we report a molecular tube with polyaromatic frameworks prepared by the Zincke cross-coupling reaction. The tube has a well-defined cylindrical cavity with a diameter and length of ~1 nm encircled by multiple anthracene panels and thereby binds long hydrocarbons containing branched methyl groups and/or unsaturated carbon–carbon double bonds (for example, heptamethylnonane, nervonic acid ester and squalene) with high selectivity in aqueous solutions. Molecules consisting of long hydrocarbon chains are of paramount importance for living organisms [1] , [2] . Phospholipids are made of fatty acids, which are long hydrocarbon chains with hydrophilic heads, and form lipid bilayers through hydrophobic and van der Waals interactions. Squalene and ubiquinones are also important biomolecules with long hydrocarbon chains containing both branched and unsaturated moieties. Within the confined nanospaces of synthetic capsule and barrel-shaped molecular hosts, long hydrocarbons can adopt unusual helical or holding conformations of the molecules [3] , [4] , [5] , [6] , [7] , [8] , [9] . However, the recognition of long hydrocarbons by synthetic hosts is a challenging task due to their conformational flexibility and the lack of distinguishing recognition sites. Thus it is not surprising that the selective binding of simple or functionalized (for example, branched methyl groups or unsaturated carbon–carbon double bonds) long hydrocarbon chains, essential components for biological function [1] , [2] , has not yet been achieved with artificial host molecules [10] , [11] , [12] , [13] , [14] . We envisioned that a tubular host providing a well-defined but open cavity encompassed with polyaromatic frameworks resembling a carbon nanobelt [15] could accomplish the selective binding of such long hydrocarbons through effective polyaromatic–aliphatic host–guest interactions ( Fig. 1a ) [16] , [17] . 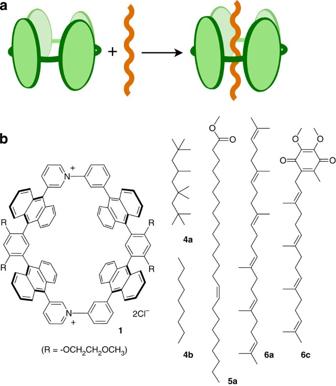Figure 1: Binding of long hydrocarbons by a polyaromatic molecular tube. (a) Schematic representation of the binding of a long hydrocarbon by a molecular tube with polyaromatic frameworks. (b) Chemical structures of molecular tube1and long hydrocarbons4a,4b,5a,6aand6c. Figure 1: Binding of long hydrocarbons by a polyaromatic molecular tube. ( a ) Schematic representation of the binding of a long hydrocarbon by a molecular tube with polyaromatic frameworks. ( b ) Chemical structures of molecular tube 1 and long hydrocarbons 4a , 4b , 5a , 6a and 6c . Full size image Herein we report the synthesis and host properties of molecular tube 1 which presents a hydrophobic cavity encircled by polyaromatic anthracene panels ( Fig. 1b ). The tube is obtained by the transition-metal-free cross-coupling reaction of end-functionalized, bent compounds with two embedded anthracene rings. The girded cylindrical cavity (~1 nm in diameter and length) of tube 1 selectively binds long hydrocarbons with branched methyl groups and/or unsaturated moieties, such as 2,2,4,4,6,8,8-heptamethylnonane ( 4a ), nervonic acid methyl ester ( 5a ), squalene ( 6a ) and coenzyme Q4 ( 6c ) ( Fig. 1b ) through hydrophobic aromatic–aliphatic and/or aromatic–olefinic interactions in 1:1 water/methanol solutions. Synthesis and characterization of molecular tube 1 We used bispyridine ligand 2b (X=non; Fig. 2a ) with two embedded anthracene panels to design molecular tube 1 . The rigidly bent conformation of 2b facilitates the formation of supramolecular assemblies such as (i) capsular structures through noncovalent, coordinative transition-metal linkages [18] , [19] , [20] , [21] and (ii) bowl-shaped structures through covalent methylene linkages [22] , [23] . For the preparation of the tubular structure, we employed Zincke reaction [24] , [25] to form two phenyl–pyridyl bonds on 1 without using a transition-metal catalyst. Zincke salt 2a (X=–C 6 H 3 (NO 2 ) 2 + ·Cl − ) was obtained from ligand 2b and subsequent Zincke reaction of 2a with diamino compound 3 gave rise to the targeted tubular assembly ( Fig. 2a ). 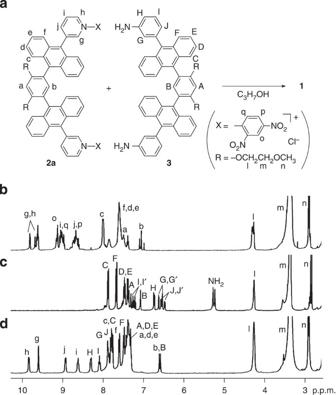Figure 2: Preparation and characterization of tube 1. (a) Schematic representation of the preparation of molecular tube1.1H NMR spectra (400 MHz, DMSO-d6, r.t.) of (b) Zincke salt2a, (c) diamine3and (d) molecular tube1. Figure 2: Preparation and characterization of tube 1. ( a ) Schematic representation of the preparation of molecular tube 1 . 1 H NMR spectra (400 MHz, DMSO- d 6 , r.t.) of ( b ) Zincke salt 2a , ( c ) diamine 3 and ( d ) molecular tube 1 . Full size image Zincke salt 2a was prepared in a moderate isolated yield (46%) in one step from bispyridine ligand 2b and 1-chloro-2,4-dinitrobenzene. In the 1 H nuclear magnetic resonance (NMR) spectrum, the pyridyl and phenyl signals ( H g–j and H o–q ) of 2a were found at considerable downfield (8.64–9.87 p.p.m. ), indicating the formation of N -phenylpyridinium units ( Fig. 2b ). When 2a and diamine 3 (ref. 26 ) were reacted in 1-propanol at 85 °C over 7 days, molecular tube 1 formed and was isolated as a yellow solid (9% yield). The 1 H NMR spectra of 2a and 3 show complicated signals for the pyridyl and phenyl rings ( Fig. 2b,c ) due to the presence of the atropisomers arising from hindered rotation around the anthryl–aryl bonds [18] . In contrast, the 1 H NMR spectrum of tube 1 revealed eight clearly resolved aromatic signals ( H g–j and H G–J ) assignable to the N -phenylpyridinium moieties between 7.86 and 9.86 p.p.m. ( Fig. 2d ). The upfield shifts of the H b and H B signals ( Δ δ=−0.4 p.p.m.) indicate a tubular structure, in which the interior aromatic protons are shielded by the adjacent anthracene panels. Electrospray ionization time-of-flight mass spectrometry (ESI-TOF MS) analysis confirmed the formation of 1 with a molecular weight of 1,532.67 Da: a prominent signal was observed at m/z =730.9, assigned to the [ 1 −2Cl − ] 2+ species. The structure of 1 was unambiguously confirmed by X-ray crystallographic analysis. Pale-yellow crystals suitable for X-ray analysis grew by slow evaporation of a methanol solution of 1 at room temperature (r.t.) for 1 week. The tube-shaped structure of 1 is ~1 nm long and is composed of four anthracene panels connected by alternating N -phenylpyridinium and phenylene spacers ( Fig. 3 ). The pyridyl–phenyl groups adopt slightly twisted conformations (average 41.6°). The open cylindrical cavity of 1 is fully girded by the polyaromatic anthracene panels with inner diagonal distances of 0.9–1.1 nm. The tubular structure provides a well-defined hydrophobic nanospace and hydrophilic pyridinium and methoxyethoxy groups so that we examined the host capability of the amphiphilic tube 1 for long hydrocarbons in aqueous solutions. 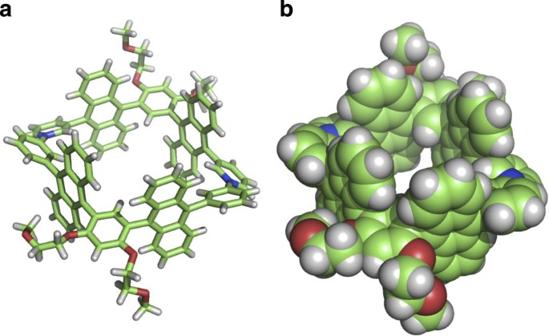Figure 3: X-ray crystal structure of tube 1. (a) Stick and (b) space-filling representations. Solvent molecules and counterions are omitted for clarity. Figure 3: X-ray crystal structure of tube 1. ( a ) Stick and ( b ) space-filling representations. Solvent molecules and counterions are omitted for clarity. Full size image Selective binding of a branched alkane Molecular tube 1 binds various n -alkanes (C n H 2 n+ 2 ) but shows selectivity for a multiply branched alkane over nonbranched alkanes. For example, when branched 2,2,4,4,6,8,8-heptamethylnonane ( 4a ; 2.2 μmol) and linear n -nonane ( 4b ; 2.2 μmol) were suspended in a 1:1 D 2 O/CD 3 OD solution (0.8 ml) of tube 1 (0.78 μmol) at room temperature for 3 h, the tube selectively bound one molecule of 4a (>98% selectively), through hydrophobic forces, to give a 1:1 host–guest 1 · 4a complex in 67% yield ( Fig. 4a ), as confirmed by NMR and MS analyses. The 1 H NMR spectrum showed the five methyl signals of 4a in the range of −0.31 to −1.13 p.p.m. ( Fig. 4b ), which are highly shifted upfield by Δ δ max =−2.08 p.p.m., due to shielding effects from the encircling anthracene rings. The 1:1 host–guest ratio was supported by ESI-TOF MS measurement, where a prominent signal was observed at m/z =843.8 corresponding to a [ 1 · 4a −2Cl − ] 2+ ion. In the crystal structure of 1 · 4a , the hydrocarbon chain of bound guest 4a is highly disordered in the cavity of 1 and cannot be located in the crystallographic analysis. Thus the structure of 4a within 1 was optimized by semiempirical calculation (PM3 level). The host–guest structure revealed that the bound alkane with branched methyl groups fully occupies the cavity of the tube with multiple CH–π interactions ( Fig. 4e ), which are also supported by the NOESY study. Linear alkanes such as 4b , n -dodecane ( 4c ) and n -hexadecane ( 4d ) were also bound by tube 1 under similar conditions to give host–guest complexes 1 · 4b , 1 · 4c and 1 · 4d (92, 46 and 12% yields, respectively). In the 1 H NMR spectra, the bound guest signals for 4b and 4d were found in the range of 0.24 to −0.16 p.p.m. ( Fig. 4c ) and −0.18 to −0.94 p.p.m. ( Fig. 4d ), respectively, with significant upfield shifts. However, competitive binding experiments revealed the binding preference of tube 1 for the branched and nonbranched alkanes to be 4a >> 4b–d ( Fig. 4a ). We hypothesize that the preferential binding of the branched hydrophobic guest stems from more efficient filling of the hydrophobic nanospace. 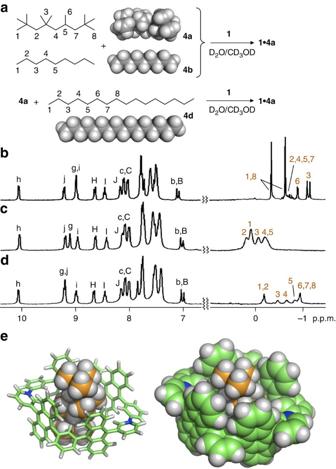Figure 4: Selective binding of a branched alkane by tube 1. (a) Schematic representation of the selective binding of 2,2,4,4,6,8,8-heptamethylnonane (4a) by molecular tube1(>98% selectivity) from a mixture of4aandn-nonane (4b) orn-hexadecane (4d) in a 1:1 D2O/CD3OD solution and (b) the resultant1H NMR spectrum (400 MHz, D2O:CD3OD=1:1, r.t.) of1·4a.1H NMR spectra (400 MHz, D2O:CD3OD=1:1, r.t.) of (c)1·4band (d)1·4d. (e) Molecular structure of1·4a: the framework of tube1is the crystal structure (substituents are omitted for clarity) and the structure of bound4ais optimized by semiempirical calculation (PM3 level). Figure 4: Selective binding of a branched alkane by tube 1. ( a ) Schematic representation of the selective binding of 2,2,4,4,6,8,8-heptamethylnonane ( 4a ) by molecular tube 1 (>98% selectivity) from a mixture of 4a and n -nonane ( 4b ) or n -hexadecane ( 4d ) in a 1:1 D 2 O/CD 3 OD solution and ( b ) the resultant 1 H NMR spectrum (400 MHz, D 2 O:CD 3 OD=1:1, r.t.) of 1 · 4a . 1 H NMR spectra (400 MHz, D 2 O:CD 3 OD=1:1, r.t.) of ( c ) 1 · 4b and ( d ) 1 · 4d . ( e ) Molecular structure of 1 · 4a : the framework of tube 1 is the crystal structure (substituents are omitted for clarity) and the structure of bound 4a is optimized by semiempirical calculation (PM3 level). Full size image Selective binding of unsaturated fatty acid esters Next we disclosed that molecular tube 1 selectively binds nervonic acid methyl ester ( 5a ), a hydrocarbon chain with a single unsaturated moiety, over lignoceric acid methyl ester ( 5b ), the fully saturated analogue ( Fig. 5a ). When a mixture of 5a and 5b (1.8 μmol each) was combined in a 1:1 D 2 O/CD 3 OD solution of tube 1 (0.78 μmol) at room temperature for 3 h, the formation of a host–guest 1 · 5a complex in 30% yield was indicated by the NMR and ESI-TOF MS analyses. In the 1 H NMR spectrum ( Fig. 5b ), the aliphatic signals of guest 5a were shifted upfield ( Δ δ>1.48 p.p.m.) after inclusion within tube 1 and appeared in the range of 0.79 to −1.49 p.p.m. The tubular framework is able to move along the long hydrocarbon chains on the NMR timescale (~0.1 s) so that proton peaks for the end of the chains were also shifted upfield. The exclusive binding of 5a by the tube (>99% selectivity) was unambiguously confirmed, because no proton signal of bound 5b was observed in the 1 H NMR spectrum after the combination of 1 and 5b in a water/methanol solution. Therefore, the tube strictly recognized the existence of a single carbon–carbon double bond within the long hydrocarbon ester, presumably through polyaromatic–olefinic host–guest interactions. 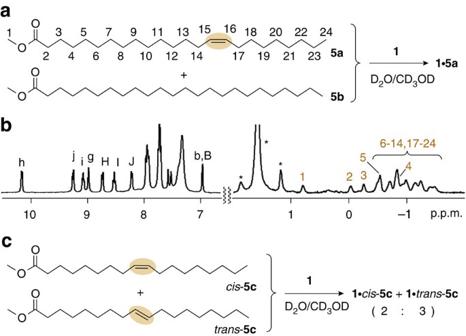Figure 5: Selective binding of unsaturated fatty acid esters by tube 1. (a) Schematic representation of the selective binding of nervonic acid methyl ester (5a) by tube1(>99% selectivity) from a mixture of5aand lignoceric acid methyl ester (5b) in a 1:1 D2O/CD3OD solution and (b) the resultant1H NMR spectrum (400 MHz, D2O:CD3OD=1:1, r.t., *=free guests). (c) Schematic representation of the binding of oleic acid methyl ester (cis-5c) and elaidic acid methyl ester (trans-5c) by tube1. Figure 5: Selective binding of unsaturated fatty acid esters by tube 1. ( a ) Schematic representation of the selective binding of nervonic acid methyl ester ( 5a ) by tube 1 (>99% selectivity) from a mixture of 5a and lignoceric acid methyl ester ( 5b ) in a 1:1 D 2 O/CD 3 OD solution and ( b ) the resultant 1 H NMR spectrum (400 MHz, D 2 O:CD 3 OD=1:1, r.t., *=free guests). ( c ) Schematic representation of the binding of oleic acid methyl ester ( cis - 5c ) and elaidic acid methyl ester ( trans - 5c ) by tube 1 . Full size image Tube 1 can bind both cis- and trans -isomers of unsaturated fatty acid esters. For instance, oleic acid methyl ester ( cis - 5c ) and elaidic acid methyl ester ( trans - 5c ) were both enclathrated by 1 to generate 1:1 host–guest complexes in 77 and 90% yields, respectively. A competitive binding experiment of 1 with a mixture of cis - 5c and trans - 5c displayed the formation of 1 · cis - 5c and 1 · trans - 5c complexes in a 2:3 ratio as thermodynamically stable products ( Fig. 5c ). Selective binding of branched and unsaturated hydrocarbons Finally, we determined the ability of tube 1 to bind long hydrocarbons containing both branches and unsaturated moieties and showed the selective binding of squalene and coenzyme Q4, bearing multiple methyl groups and unsaturated carbon–carbon double bonds, by 1 in aqueous solutions, due to the synergistic effect of hydrophobic aromatic–aliphatic and aromatic–olefinic interactions. When tube 1 , squalene ( 6a ) and squalane ( 6b ), which is the fully hydrogenated squalene, were combined in a 1:1 D 2 O/CD 3 OD solution, the tube bound squalene with high selectivity (>99%) at room temperature to afford a 1 · 6a complex (24% yield), as confirmed by NMR analysis ( Fig. 6a,b ). The size and shape of 6b are comparable to that of 6a , but surprisingly 6b was not bound at all by 1 even in the absence of 6a . 1 H NMR spectrum of 1 · 6a displayed significant upfield shifts of the signals corresponding to the methyl and methylene moieties of 6a ( Fig. 6b ). Proton signals for the methyl groups ( H 10 and H 6 ) and the methylene units ( H 8 and H 9 ) appeared around −0.54 p.p.m. and −0.22 p.p.m., respectively, with huge upfield shifts ( Δ δ=2.2 p.p.m. ), indicating tight contacts between the central part of 6a and the anthracene frameworks of 1 . The NOESY NMR spectrum showed several sets of correlation signals between the tube and the bound guest (for example, H B,b – H 10 , H C,c – H 10 and H F,f – H 8,9 ). An optimized structure of 1′ · 6a (R=H), which is in good agreement with the NOESY study, shows that the long hydrocarbon chain (2.7 nm in diameter) of 6a is partially sandwiched by the anthracene panels of 1 ( Fig. 5c ). Furthermore, we note that tube 1 binds coenzyme Q4 ( 6c ), composed of a branched and unsaturated hydrocarbon chain and a benzoquinone moiety, to give rise to a 1 · 6c complex in 61% yield under similar conditions. 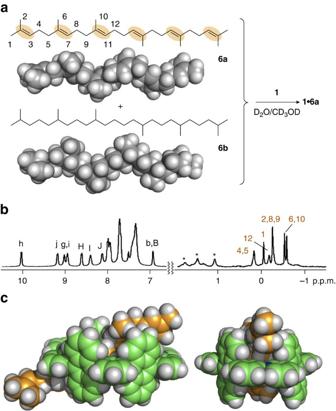Figure 6: Selective binding of a branched and unsaturated hydrocarbon by tube 1. (a) Schematic representation of the selective binding of squalene (6a) by tube1(>99% selectivity) from a mixture of6aand squalane (6b) in a 1:1 D2O/CD3OD solution and (b) the resultant1H NMR spectrum (400 MHz, D2O:CD3OD=1:1, r.t., *=free guests). (c) Optimized structure of1′·6a(R=H, semiempirical calculation, PM3 level). Figure 6: Selective binding of a branched and unsaturated hydrocarbon by tube 1. ( a ) Schematic representation of the selective binding of squalene ( 6a ) by tube 1 (>99% selectivity) from a mixture of 6a and squalane ( 6b ) in a 1:1 D 2 O/CD 3 OD solution and ( b ) the resultant 1 H NMR spectrum (400 MHz, D 2 O:CD 3 OD=1:1, r.t., *=free guests). ( c ) Optimized structure of 1′ · 6a (R=H, semiempirical calculation, PM3 level). Full size image In this study, we demonstrated for the first time the selective recognition and binding of long linear, branched and unsaturated hydrocarbons by a synthetic tubular host. The tube has a well-defined and open cylindrical cavity (~1 nm) encircled by multiple polyaromatic panels. The girding polyaromatic panels encompass long hydrocarbon chains with diameters of ~1–3 nm through effective hydrophobic aromatic–aliphatic and/or aromatic–olefinic interactions in aqueous solutions. The present studies show a new strategy for recognizing and sensing various long and flexible hydrocarbons (for example, essential biomolecules) by polyaromatic tubular nanospace. General NMR: Bruker AVANCE-400 (400 MHz) and AVANCE-HD500 (500 MHz), ESI-TOF MS: Bruker micrOTOF II, FT-IR: JASCO FT/IR-4200, X-ray: Bruker APEXII ULTRA/CCD diffractometer, GPC: JAI LC-9225NEXT, elemental analysis: LECO CHNS-932 VTF-900. Solvents and reagents: TCI Co., Ltd., WAKO Pure Chemical Industries Ltd., KANTO CHEMICAL CO., INC., Sigma-Aldrich Co. and Cambridge Isotope Laboratories, Inc. Bispyridine ligand 2b and diamine 3 were synthesized according to previously reported procedures [18] , [26] . Synthesis of Zincke salt 2a Bispyridine ligand 2b (951.7 mg, 1.298 mmol), 1-chloro-2,4-dinitorobenzene (3.263 g, 16.11 mmol) and methanol (60 ml) were added to a 100 ml glass flask. The mixture was stirred at 67 °C for 3 weeks and then concentrated under reduced pressure. The crude product was washed with diethyl ether, acetone and CHCl 3 to afford Zincke salt 2a as a yellow solid (632.5 mg, 592.7 μmol, 46% yield; See Supplementary Figs 1 and 2 ). 1 H NMR (400 MHz, DMSO- d 6 , r.t.): δ 9.84 (d, J =4.8 Hz, 1H), 9.71–9.63 (m, 3H), 9.18–9.14 (m, 2H), 9.10–8.98 (m, 4H), 8.78–8.64 (m, 4H), 8.02 (d, J =5.3 Hz, 4H), 7.87 (br, 2H), 7.63–7.47 (m, 10H), 7.42–7.38 (m, 1H), 7.11–7.00 (m, 1H), 4.30–4.25 (m, 4H), 3.44 (m, 4H), 2.89–2.84 (m, 6H). 13 C NMR (100 MHz, DMSO- d 6 , r.t.): δ 158.0 (C q ), 151.2 (C q ), 149.2 (CH), 147.1, 145.7 (CH), 143.1 (CH), 138.7 (C q ), 138.3 (C q ), 136.2 (CH), 132.0, 130.2, 129.7, 128.6, 127.0, 125.8, 121.3, 118.3, 99.8 (CH), 70.2 (CH 2 ), 70.1 (CH 2 ), 68.2 (CH 2 ), 68.0 (CH 2 ), 57.9 (CH 3 ), 57.9 (CH 3 ). FT-IR (KBr, cm −1 ): 3,397, 3,060, 2,928, 2,883, 2,828, 1,607, 1,572, 1,541, 1,495, 1,442, 1,384, 1,343, 1,314, 1,266, 1,194, 1,160, 1,125, 1,083, 1,053, 1,027, 912, 836, 770, 739, 689. HR MS (ESI-TOF; CH 3 OH): m/z Calcd. 533.1581, Found 533.1581 [ 2a −2Cl − ] 2+ . Synthesis of tube 1 Zincke salt 2a (600.4 mg, 0.5276, mmol), diamine 3 (416.1 mg, 0.5247, mmol) and 1-propanol (300 ml) were added to a 500 ml glass flask. The mixture was stirred at 85 °C for 7 d and then concentrated under reduced pressure. The crude product was washed with diethyl ether. A mixed solution of CHCl 3 , hexane, DMSO and water was added to the crude product and then the aqueous phase was collected. The crude product in the aqueous solution was extracted with CHCl 3 . After evaporation, the resultant solid was purified by GPC to afford tube 1 as a yellow solid (72.7 mg, 47.4 μmol, 9% yield; See Supplementary Figs 3–9 ). Pale-yellow single crystals suitable for X-ray crystallographic analysis were obtained by slow evaporation of a CH 3 OH solution of tube 1 at room temperature for 1 week ( Supplementary Figs 10 and 11 , Supplementary Table 1 and Supplementary Data 1 ). 1 H NMR (400 MHz, DMSO- d 6 , r.t.): δ 9.86 (d, J =6.4 Hz, 2H), 9.62 (s, 2H), 8.95 (d, J =7.6 Hz, 2H), 8.64 (dd, J =6,4, 7.6 Hz, 2H), 8.32 (d, J =8.2 Hz, 2H), 8.10 (dd, J =7.6, 8.2 Hz, 2H), 7.90–7.80 (m, 12H), 7.61 (d, J =8.8, 4H), 7.49 (d, J =8.4, 4H), 7.46–7.33 (m, 18H), 6.61 (s, 1H), 6.58, (s, 1H), 4.27–4.23 (m, 8H), 3.35–3.33 (m, 8H), 2.90 (s, 6H), 2.87 (s, 6H). 13 C NMR (100 MHz, DMSO- d 6 , r.t.): δ 157.9 (C q ), 157.8 (C q ) 148.7 (CH), 145.4 (CH), 143.9 (CH), 142.6 (C q ), 140.1 (C q ), 138.7 (C q ), 135.3 (CH), 133.8 (C q ), 133.5 (CH), 130.3 (CH), 129.5 (C q ), 129.3 (C q ), 129.0 (C q ), 128.3 (CH), 127.8 (C q ), 127.4 (CH), 126.5 (CH, C q ), 126.2 (C q ), 126.0 (CH), 125.8 (CH), 125.5 (CH), 125.1(C q ), 123.6 (CH), 118.6 (C q ), 118.2 (C q ), 99.7 (CH), 70.1 (CH 2 ), 68.0 (CH 2 ), 57.8 (CH 3 ). DOSY NMR (400 MHz, DMSO- d 6 , 300 K): D =2.73 × 10 −10 m 2 s −1 . FT-IR (KBr, cm −1 ): 3,410, 3,062, 2,978, 2,926, 2,883, 2,817, 1,604, 1,573, 1,504, 1,443, 1,383, 1,358, 1,311, 1,266, 1,195, 1,155, 1,124, 1,130, 1,054, 1,029, 944, 808, 770, 688, 611. ESI-TOF MS (CH 3 OH): m/z Calcd. 730.8, Found 730.9 [ 1 –2Cl − ] 2+ . E.A. : Calcd. for C 102 H 80 O 8 N 2 Cl 2 ·H 2 O· 1.5CHCl 3 : C, 71.87; H, 4.87; N, 1.62, Found: C, 71.87; H, 4.69; N, 1.67. Binding of heptamethylnonane by tube 1 2,2,4,4,6,8,8-Heptamethylnonane ( 4a ; 0.71 mg, 3.1 μmol) was added to a D 2 O:CD 3 OD solution (1:1 (v/v), 0.3 ml) of 1 (1.2 mg, 0.78 μmol) and the mixture was stirred at r.t. for 3 h. The formation of a 1 · 4a complex was confirmed by NMR and ESI-TOF MS analyses ( Supplementary Figs 12–15 ). The product yield (91%) was estimated by 1 H NMR analysis. Pale-yellow single crystals suitable for X-ray crystallographic analysis were obtained at room temperature for 3 days after the addition of NaCl (a few grains) to a H 2 O/CH 3 OH solution of 1 · 4a ( Supplementary Figs 16 and 17 and Supplementary Table 2 ). Similarly, 1 · 4b–e complexes were obtained under the similar conditions ( Supplementary Methods , Supplementary Figs 18–27 and Supplementary Data 2 ). 1 H NMR (400 MHz, D 2 O:CD 3 OD=1:1, r.t.): δ 10.02 (d, J =6.4 Hz, 2H), 9.19 (d, J =7.2 Hz, 2H), 8.98–8.96 (m, 4H), 8.62 (d, J =8.8 Hz, 2H), 8.43 (dd, J =8.8, 8.0 Hz, 2H),, 8.15 (d, J =8.0 Hz, 2H), 8.14–8.02 (m, 8H), 7.80–7.49 (m, 28H), 7.14 (s, 1H), 7.09 (s, 1H), 4.47 (br, 8H), 3.65 (br, 8H), 3.05–3.03 (m, 12H), −0.30 (s, 4a ), −0.57 (s, 4a ), −0.62–0.71 (m, 4a ), −0.85 (d, J =6.4 Hz, 4a ) −1.04 (s, 4a ), −1.09 (s, 4a ). ESI-TOF MS (H 2 O:CH 3 OH=1:1): m/z Calcd. 843.9, Found 843.8 [ 1 · 4a −2Cl − ] 2+ . Binding of nervonic acid methyl ester by tube 1 Nervonic acid methyl ester ( 5a ; 1.0 mg, 2.6 μmol) was added to a D 2 O:CD 3 OD solution (1:1 (v/v), 0.4 ml) of tube 1 (0.60 mg, 0.39 μmol) and the mixture was stirred at r.t. for 3 h. The formation and yield of a 1 · 5a complex (50%) was estimated by 1 H NMR analysis ( Supplementary Fig. 28 ). Binding experiments of 5b and 5c by tube 1 were examined under the similar conditions ( Supplementary Methods and Supplementary Figs 29 and 30 ). 1 H NMR (500 MHz, D 2 O:CD 3 OD=1:1, r.t.): δ 10.18 (d, J =5.6 Hz, 2H), 9.25 (d, J =7.6 Hz, 2H), 9.10 (dd, J =5.6, 7.6 Hz, 2H), 8.93 (s, 2H), 8.76 (d, J =8.0 Hz, 2H), 8.54 (dd, J =8.0, 6.8 Hz, 2H), 8.22 (d, J =6.8 Hz, 2H), 7.89–7.28 (m, 36H), 6.96 (s, 1H), 6.93 (s, 1H), 4.49–4.46 (m, 8H), 3.64–3.62 (m, 8H), 3.03–3.00 (m, 12H), 0.69 (br, 5a ), −0.12 (br, 5a ), −0.31 (br, 5a ), −0.61 (br, 5a ), −0.76 (br, 5a ), −0.92 (br, 5a ), −1.05 (br, 5a ), −1.12 (br, 5a ), −1.15 (br, 5a ), −1.24 (br, 5a ), −1.34 (br, 5a ). Binding of squalene by tube 1 Squalene ( 6a ; 0.16 mg, 0.38 μmol) was added to a D 2 O:CD 3 OD solution (1:1 (v/v), 0.4 ml) of tube 1 (0.60 mg, 0.39 μmol) and the mixture was stirred at r.t. for 3 h. The solution was estimated by 1 H NMR analysis ( Supplementary Figs 31–33 ). The formation and yield of a 1 · 6a complex (36%) was estimated by 1 H NMR analysis. Binding experiments of 6b and 6c by tube 1 were examined under the similar conditions ( Supplementary Methods and Supplementary Figs 34 and 35 ). 1 H NMR (400 MHz, D 2 O:CD 3 OD=1:1, r.t.): δ 10.07 (d, J =6.4 Hz, 2H), 9.24 (d, J =8.0 Hz, 2H), 9.02–8.98 (m, 4H), 8.67 (d, J =8.0 Hz, 2H), 8.47 (dd, J =8.0, 7.6 Hz, 2H), 8.22 (d, J =7.6 Hz, 2H), 8.06–8.00 (m, 8H), 7.83–7.75 (m, 10H), 7.59 (s, 1H), 7.52 (s, 1H), 7.43 (br, 16H), 7.00 (s, 1H), 6.99 (s, 1H), 4.51–4.47 (m, 8H), 3.67 (br, 8H), 3.06–3.03 (m, 12H), 2.90 (br, 6a ), 2.68 (br, 6a ), 0.24 (br, 6a ), 0.04 (br, 6a ), −0.10 (br, 6a ), −0.17 (br, 6a ), −0.47 (br, 6a ), −0.52 (br, 6a ). Competitive binding experiment of 4a and 4b by 1 Alkanes 4a (0.50 mg, 2.2 μmol) and 4b (0.28 mg, 2.2 μmol) were added to a D 2 O:CD 3 OD solution (1:1 (v/v), 0.8 ml) of tube 1 (1.2 mg, 0.78 μmol) and then the mixture was stirred at r.t. for 3 h. After the organic phase including excess guests was removed by centrifugation, the aqueous phase was collected. The selective formation of host–guest complex 1 · 4a (>98% selectivity, 67% yield) was confirmed by the 1 H NMR and GC–MS analyses of the resultant aqueous solution (See Supplementary Figs 36 and 37 ). Competitive binding experiments of 4a versus 4c and 4a versus 4d by tube 1 were examined under the similar conditions (See Supplementary Methods and Supplementary Figs 38 and 39 ). Competitive binding experiment of 5a and 5b by 1 Fatty acid esters 5a (0.69 mg, 1.8 μmol) and 5b (0.70 mg, 1.8 μmol) were added to a D 2 O:CD 3 OD solution (1:1 (v/v), 0.8 ml) of tube 1 (1.2 mg, 0.78 μmol) and then the mixture was stirred at r.t. for 3 h. After the excess guests were removed by centrifugation, the selective formation of host–guest complex 1 · 5a (>99% selectivity, 30% yield) was confirmed by the 1 H NMR and ESI-TOF MS analyses of the resultant aqueous phase ( Supplementary Fig. 40 ). Competitive binding experiments of cis - 5c and trans - 5c by tube 1 were examined under the similar conditions (See Supplementary Methods and Supplementary Figs 41 and 42 ). Competitive binding experiment of 6a and 6b by 1 A mixture of squalene ( 6a ; 2.0 mg, 4.9 μmol) and squalane ( 6b ; 2.0 mg, 4.7 μmol) was added to a D 2 O:CD 3 OD solution (1:1 (v/v), 0.8 ml) of tube 1 (3.2 mg, 2.1 μmol) and the mixture was stirred at r.t. for 3 h. After the excess guests were removed by centrifugation, the selective formation of host–guest complex 1 · 6a (>99% selectivity, 24% yield) was confirmed by the 1 H NMR analysis of the resultant aqueous phase (See Supplementary Figs 43 and 44 ). Accession codes : CCDC-977769 and 996970 contain the supplementary crystallographic data for the structures reported in this article. These data can be obtained free of charge from The Cambridge Crystallographic Data Centre (CCDC) via www.ccdc.cam.ac.uk/data_request/cif . How to cite this article: Yazaki, K. et al. A polyaromatic molecular tube that binds long hydrocarbons with high selectivity. Nat. Commun. 5:5179 doi: 10.1038/ncomms6179 (2014).